Transparent air filter for high-efficiency PM2.5capture Particulate matter (PM) pollution has raised serious concerns for public health. Although outdoor individual protection could be achieved by facial masks, indoor air usually relies on expensive and energy-intensive air-filtering devices. Here, we introduce a transparent air filter for indoor air protection through windows that uses natural passive ventilation to effectively protect the indoor air quality. By controlling the surface chemistry to enable strong PM adhesion and also the microstructure of the air filters to increase the capture possibilities, we achieve transparent, high air flow and highly effective air filters of ~90% transparency with >95.00% removal of PM 2.5 under extreme hazardous air-quality conditions (PM 2.5 mass concentration >250 μg m −3 ). A field test in Beijing shows that the polyacrylonitrile transparent air filter has the best PM 2.5 removal efficiency of 98.69% at high transmittance of ~77% during haze occurrence. Particulate matter (PM) pollution in air affects people’s living quality tremendously, and it poses a serious health threat to the public as well as influencing visibility, direct and indirect radiative forcing, climate, and ecosystems [1] , [2] , [3] , [4] , [5] , [6] , [7] . PM is a complex mixture of extremely small particles and liquid droplets [1] , [8] . On the basis of the particle size, PM is categorized by PM 2.5 and PM 10 , which refer to particle sizes below 2.5 and 10 μm, respectively. PM 2.5 pollution is particularly harmful since it can penetrate human bronchi and lungs owing to the small particle size [9] . Hence, long-term exposure to PM 2.5 increases morbidity and mortality [10] , [11] , [12] , [13] , [14] . Recently, there have been serious PM pollution problems in developing countries with a large manufacturing industry such as China. 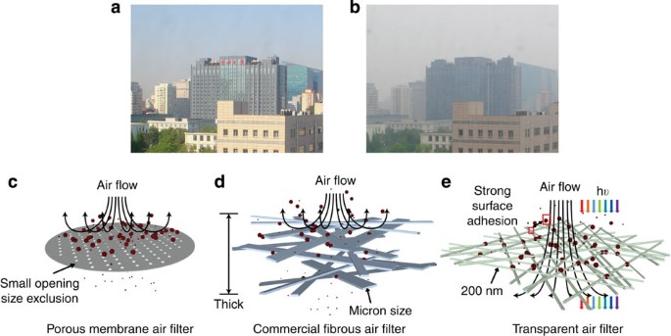Figure 1: Particulate matter pollution and comparison among different air filters. (a) Photograph of a random place in Beijing during a sunny day. (b) Photograph of the same place in Beijing during a hazy day with hazardous PM2.5level. (c) Schematics of porous air filter capturing PM particles by size exclusion. (d) Schematics of bulky fibrous air filter capturing PM particles by thick physical barrier and adhesion. (e) Schematics of transparent air filters that capture PM particles by strong surface adhesion and allowing a high light and air penetration. Figure 1a,b shows images of a location in Beijing during clear and hazy days, respectively. During hazy days, the visibility decreased greatly and the air quality was poor because of extremely high levels of PM 2.5 . Figure 1: Particulate matter pollution and comparison among different air filters. ( a ) Photograph of a random place in Beijing during a sunny day. ( b ) Photograph of the same place in Beijing during a hazy day with hazardous PM 2.5 level. ( c ) Schematics of porous air filter capturing PM particles by size exclusion. ( d ) Schematics of bulky fibrous air filter capturing PM particles by thick physical barrier and adhesion. ( e ) Schematics of transparent air filters that capture PM particles by strong surface adhesion and allowing a high light and air penetration. Full size image Measures taken by the public during hazy days are mostly focused on outdoor individual protection, such as using mask filters, which are often bulky and resistant to air flow [15] . In indoor spaces, protection is only available in modern commercial buildings through filtering in ventilation systems or central air conditioning; residential housing seldom has filtration protection from PM. Moreover, all these active air exchanges by mechanical ventilation consume enormous amounts of energy because of the massive use of pumping systems [16] . When people stay indoors without sufficient air exchange, indoor air quality is also of great concern [17] . It would be ideal if passive air exchange—that is, natural ventilation—through windows could be used for indoor air filtration. Owing to the large surface area of most windows, air exchange is very efficient. Protection at windows requires the air filters to not only possess a high PM-capture ability but also a high optical transparency for natural lighting from the sun and sight-viewing at the same time. Here we introduce the concept of a transparent air filter for indoor air-quality protection at the window for the first time. The PM 2.5 pollution particles in air have complicated compositions including inorganic matter (such as SiO 2 , SO 4 2− and NO 3 − ) and organic matter (such as, organic carbon and elemental carbon) from diverse sources including soil dust, vehicular emission, coal combustion, secondary aerosols, industrial emission and biomass burning [1] , [18] , [19] , [20] , [21] . The behaviour of PM particles are different because of their chemical compositions, morphologies and mechanical properties [15] . Some rigid inorganic PM particles are mainly captured by interception and impaction on a filter surface. Some soft PM containing a lot of carbon compounds or water such as those from combustion exhaust would deform on filter surfaces and require stronger binding during the process of attaching to the filter. It is important to study the surface properties of the air filters to enhance PM particle capture. However, in existing air filter technology, not much work has been performed to study the properties of filter materials. There are two types of air filters in common use [15] . One is a porous membrane filter, which is similar to a water filtration filter (shown in Fig. 1c ). This type of air filter is made by creating pores on solid substrate, and it usually has very small pore size to filter out PM with larger sizes and the porosity of this type of filter is low (<30%). Hence, the filtration efficiency is high, although the pressure drop is large. Another type of air filter is a fibrous air filter, which captures PM particles by the combination of thick physical barriers and adhesion (shown in Fig. 1d ). This type of filter usually has porosities >70% and is made of many layers of thick fibres of diverse diameters from several microns to tens of microns. To obtain a high efficiency, this type of filter is usually thick. The deficiency of the second type of filter is the bulkiness, nontransparency and the compromise between air flow and filter efficiency. Existing technology would not meet the requirements of a transparent high-efficiency PM 2.5 filter. Here we demonstrate a novel polymer nanofibre filter technology, which has attractive attributes of high filtering efficiency, good optical transparency, low resistance to air flow and light weight as shown in Fig. 1e . We found that when the surface chemistry of the air filter is optimized to match that of PM particles, that the single fibre capture ability becomes much more than the existing fibrous filters. Therefore, the material use in the air filter can be reduced significantly to a transparent level to enable both transparency to sunlight and sufficient air flow. In addition, when the fibre diameter is decreased to the nanometre scale, with the same packing density, the particle-capture possibility is increased a lot because of large surface area, which also ensures effective PM capture with a much thinner air filter. This transparent filter can be applied to all types of situations including personal masking and building windows. By controlling the surface chemistry and microstructure of the air filters, we report transparent ultrathin filters of ~90% transparency with >95.00% removal, of ~60% transparency with >99.00% removal and ~30% transparency with >99.97% removal of PM 2.5 particles under extreme hazardous air-quality condition. Transparent air filter surface screening To find the most effective material for transparent air filters, different polymers and polymers with other coatings were investigated for PM capture. Electrospinning was used to make polymer nanofibrous air filters (shown in Fig. 2a ). Electrospinning has great advantages in making uniform fibrous filters from diverse polymer solutions with controllable dimensions [22] , [23] , [24] , [25] . This versatility makes electrospinning an ideal tool to produce a transparent nanofibre network [26] , [27] . During electrospinning, a high voltage is applied to the tip of a syringe containing a polymer solution; the resulting electrical force pulls the polymer solution into a nanofibre and deposits the fibre on a grounded collector, which in this experiment was a commercial metal-coated window screen mesh. Owing to the electrical field distribution, the electrospun polymer nanofibres lie across the mesh holes and form network for air filtration. This electrospinning method is scalable and with the window screen as a supporting and adhering substrate, the air filter is mechanically robust. Nanofibres with different surface properties are made by changing the functional groups on the polymer side chains and also by coating different materials using a sputtering method. The chosen polymers are available in large quantity and at low cost, including polyacrylonitrile (PAN), polyvinylpyrrolidone (PVP), polystyrene (PS), polyvinyl alcohol (PVA) and polypropylene (PP). The coating materials are copper and carbon. PP, copper and carbon are all commonly used materials in commercial fibrous or porous membrane air filters [15] . The molecular models and formulae of the different polymers are shown in Fig. 2b . The polarity and hydrophobicity are different between each polymer and the dipole moments are 3.6, 2.3, 0.7, 1.2 and 0.6 D for the repeating units of PAN, PVP, PS, PVA and PP, respectively. 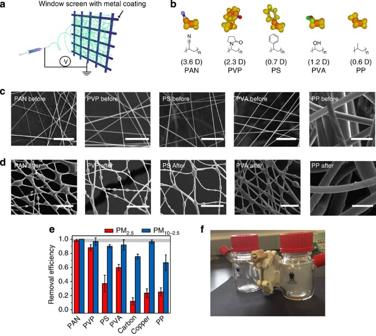Figure 2: Performance of PM2.5capture by transparent air filters with different surfaces. (a) Schematics showing the fabrication of transparent air filter by electrospinning. (b) Molecular model and formula of different polymers including PAN, PVP, PS, PVA and PP with calculated dipole moments of the repeating units of each polymer. (c) SEM images of PAN, PVP, PS, PVA and PP transparent filters before filtration. (d) SEM images of PAN, PVP, PS, PVA and PP transparent filters after filtration showing the PM attachment. Scale bars inc,d, 5 μm. (e) Removal efficiency comparison between PAN, PVP, PS, PVA, PP carbon and copper transparent filters with same fibre diameter of ~200 nm and same transmittance of ~70%. Error bar represents the standard deviation of three replicate measurements. (f) Demonstration of using transparent filter to shut off PM from the outdoor (right bottle) from entering the indoor (left bottle) environment. Figure 2: Performance of PM 2.5 capture by transparent air filters with different surfaces. ( a ) Schematics showing the fabrication of transparent air filter by electrospinning. ( b ) Molecular model and formula of different polymers including PAN, PVP, PS, PVA and PP with calculated dipole moments of the repeating units of each polymer. ( c ) SEM images of PAN, PVP, PS, PVA and PP transparent filters before filtration. ( d ) SEM images of PAN, PVP, PS, PVA and PP transparent filters after filtration showing the PM attachment. Scale bars in c , d , 5 μm. ( e ) Removal efficiency comparison between PAN, PVP, PS, PVA, PP carbon and copper transparent filters with same fibre diameter of ~200 nm and same transmittance of ~70%. Error bar represents the standard deviation of three replicate measurements. ( f ) Demonstration of using transparent filter to shut off PM from the outdoor (right bottle) from entering the indoor (left bottle) environment. Full size image In this study, the PM is generated by burning incense. The burning incense contains PM above 45 mg g −1 burned, and the exhaust smoke contains a variety of pollutant gases, including CO, CO 2 , NO 2 , SO 2 and also volatile organic compounds, such as benzene, toluene, xylenes, aldehydes and polycyclic aromatic hydrocarbons [28] . This complex air exhaust is a model system containing many of the components present in polluted air during hazy days. A scanning electron microscope (SEM) was first used to characterize different fibrous filters before and after filtration. The images are shown in Fig. 2c,d . The as-made nanofibre filters of different polymers had similar morphology with fibre sizes ~200 nm and similar packing density. Since PP fibres cannot be made by electrospinning, we peeled them off from commercial mask to a transmittance of 70%. The PP thus has a different morphology, with fibres of much larger diameter as compared with the electrospun nanofibres. The SEM images of different filters after the filtration test show that the number and size of PM particles coated on the PAN filter were both larger than that of other polymers. The smoke PM formed a coating layer strongly wrapped around each nanofibre instead of only attaching to the surface of the nanofibres as in the case of inorganic PM (shown in Supplementary Fig. 1 ). For the commercial PP air filters, the PM particles captured can hardly be seen. The quantified PM 2.5 and PM 10–2.5 removal by different fibrous filters is shown in Fig. 2e . All fibrous filters are at the same transmittance (~70%). From the efficiency comparison, it is shown that the PAN has the highest removal of both PM 2.5 and PM 10–2.5 followed by PVP, PVA, PS, PP, copper and carbon. The highlighted zone (95–100%) in Fig. 2e marks the standard for a high-efficiency filter and of those tested, only the transparent PAN filter meets this requirement. The removal efficiencies are calculated by comparing the PM particle number concentration with and without air filters. The size distribution of source PM was shown in Supplementary Fig. 2 . The results showed that the polymer capture efficiencies increase with increasing dipole moment of the polymer-repeating units, suggesting that a dipole–dipole or induced-dipole force can greatly enhance the binding of PM to the polymer surface, and polymers with higher dipole moment would have better removal efficiencies of PM particles. With the same filter transmittance (packing density), PAN transparent filter showed the highest removal of both PM 2.5 (98.11±1.41%) and PM 10–2.5 (99.31±0.08%) and only PAN transparent filter qualified the high-efficiency standard of >95% removal. This means that the surface property of PAN is much better than that of PVP, PS, PVA, PP, carbon or metal surface; hence, it can ensure a higher single fibre capture ability. Inorganic PM 2.5 and PM 10–2.5 also showed that PAN air filter was most effective in capturing PM particles. The soft PM with larger amounts of carbon and water content tends to be more difficult to capture than rigid inorganic PM, since the capture efficiencies of fibrous filters made from the same material are lower in soft PM capture ( Supplementary Fig. 1 ). Besides surface chemistry, the filter’s fibre dimension also affects the PM removal efficiency significantly as shown in Supplementary Fig. 3 . As the fibre diameter increased from ~200 nm to ~1 μm, the removal efficiencies of PAN air filters with the same transmittance of 70% decreased dramatically from 98.11±1.41% to 48.21±4.19%. A demonstration of using a transparent filter to block PM pollution was shown in Fig. 2f . In the right bottle, a hazardous level of PM with PM 2.5 index >300 or PM 2.5 mass concentration >250 μg m −3 was generated and a PAN transparent filter with ~70% transmittance was placed between the PM source and another bottle. As shown in Fig. 2f , the left bottle was still clear and the PM 2.5 concentration was in a good level marked by the PM 2.5 index (mass concentration <15 μg m −3 ). This demonstration shows the excellent efficacy of the PAN transparent filter. Performance of transparent air filter Besides capture efficiency, the other two important parameters for a transparent air filter, light transmittance and air flow, were then evaluated. 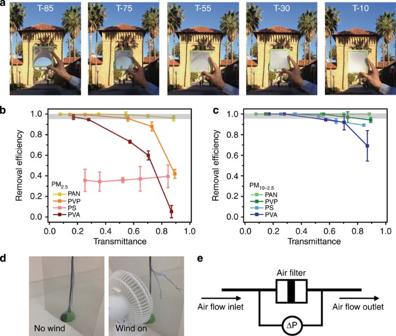Figure 3: Transparency and air flow evaluation of transparent air filters. (a) Photographs of PAN transparent air filters at different transparency. (b) PM2.5removal efficiencies of PAN, PVP, PS, PVA transparent filters at different transmittances. (c) PM10–2.5removal efficiencies of PAN, PVP, PS and PVA transparent filters at different transmittances. Error bar represents the standard deviation of three replicate measurements. (d) Photograph showing that the transparent filter can enable efficient air exchange demonstrated by an electric fan at wind velocity of 3m s−1. (e) Schematics showing the set-up for the measurement of pressure drop of air filters. Figure 3a shows the photographs of the PAN transparent air filters with transmittance of ~85, ~75, ~55, ~30 and ~10%. For the air filters with transmittance above 50%, sufficient light can penetrate through and enable lighting from sun and sight-viewing. The PM capture efficiencies of different polymer nanofibrous filters were assessed at different transmittance levels, and the results are shown in Fig. 3b,c . By increasing the thickness of the fibrous filter, the PM 2.5 capture efficiencies of PAN, PVP and PVA filters increased (shown in Fig. 3b,c ). For the PAN filter, excellent capture efficiencies were achieved for a variety of optical transmittance levels: >95.00% removal at ~90% transmittance and >99.00% removal at ~60% transmittance for PM 2.5 capture. Removal efficiencies categorized by particles size are shown in Supplementary Fig. 4 using PAN transparent filter with different transmittance. A >95.00% efficiency of PM 2.5 capture by PVP and PVA filters was achieved at lower transmittance of ~60 and ~30%, respectively. However, for PS fibres used in many commercial filters, increasing the filter thickness does not improve the PM 2.5 capture efficiency by much. The removal efficiency of PM 10–2.5 particles ( Fig. 3c ) are all higher than that of PM 2.5 in all four polymer air filters and most of the cases the removal efficiencies meet the >95.00% efficiency standard. Still, PAN showed the best capture ability than other polymer filters with similar transmittance. Figure 3: Transparency and air flow evaluation of transparent air filters. ( a ) Photographs of PAN transparent air filters at different transparency. ( b ) PM 2.5 removal efficiencies of PAN, PVP, PS, PVA transparent filters at different transmittances. ( c ) PM 10–2.5 removal efficiencies of PAN, PVP, PS and PVA transparent filters at different transmittances. Error bar represents the standard deviation of three replicate measurements. ( d ) Photograph showing that the transparent filter can enable efficient air exchange demonstrated by an electric fan at wind velocity of 3m s −1 . ( e ) Schematics showing the set-up for the measurement of pressure drop of air filters. Full size image Besides capture efficiency, keeping a high air flow is another important parameter to assess the performance of an air filter. All air flow tests were based on PAN air filter that showed the best performance in PM capture. In Fig. 3d , the air penetration through PAN transparent air filters was demonstrated by wind generated by a fan at a velocity of 3 m s −1 . A PAN transparent air filter with transmittance of ~90% was placed in front of a bundle of paper tassels hanging on a stick. When wind was blowing from the fan, the paper tassels were blown up with the PAN air filters in front of it, which demonstrated great penetration of air through the transparent filter. Quantitative analysis of the air penetration was carried out by investigating the pressure drop (Δ P ) of the transparent PAN filter with different levels of transmittance. Figure 3e shows the schematic of the pressure drop measurement. The pressure difference across the air filter was measured. It is shown in Table 1 that at a face velocity of 0.21 m s −1 , the pressure drops of 85% and 75% transmittance air filters are only 133 and 206 Pa, respectively. This pressure drop is only <0.2% of atmosphere pressure, which is negligible. These levels of pressure drop are similar to that of a blank window screen without nanofibres (131 Pa). The Δ P increases with the increase in filter thickness or the decrease in transmittance. The overall performance of the air filter considering both efficiency and pressure drop is assessed by quality factor (QF; shown in Table 1 and Supplementary Table 1 ). The transparent PAN filter showed higher QF than the four commercial filters (SEM shown in Supplementary Fig. 5 ) from twofold to even orders of magnitudes. Table 1 Performance summary of transparent air filters compared with commercial air filters. Full size table In situ time evolution study of PM capture The PM capture process and mechanism was studied by in situ optical microscope (OM) and SEM using a PAN nanofibrous filter with a fibre diameter of ~200 nm. The PAN nanofibrous filter was placed under the OM. Continuous flow with high concentration of smoke PM was fed to the fibrous filter. The dynamic process is shown in the Supplementary Movie 1 . 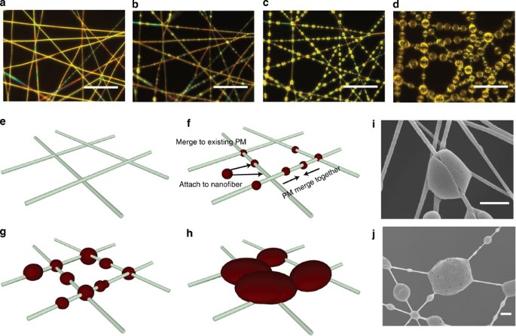Figure 4:In situtime evolution study of PM capture by PAN transparent filter. (a–d)In situstudy of PM capture by PAN nanofibre characterized by OM showing filter morphologies at different time sequences during a continuous feed. Scale bars, 20 μm. The timescales for (a–d) is 0, 5, 120 and 600 s, respectively. (e–h) Schematics showing the mechanism of PM capture by nanofibrous filter at different time sequences. (i) SEM image showing the detailed morphologies of attached soft PM that formed a coating layer wrapping around the PAN nanofibre. Scale bar, 1 μm. (j) SEM image showing that the nanofibre junction has more PM aggregated to form bigger particles. Scale bar, 1 μm. Figure 4a shows the PAN fibre filter before capturing PM. In Fig. 4b–d , the time sequence (5, 120 and 600 s) of PM capture is shown. Schematics explaining the PM capture at different stages are shown in Fig. 4e–h . At the initial capture stage ( Fig. 4b,f ), PM was captured by the PAN nanofibres and bound tightly on the nanofibres. As more smoke was fed continuously to the filter, more PM particles were attached. The particles were able to move along the PAN nanofibres and aggregate to form larger particles and left behind some empty spaces for new PM particles to attach (shown in Supplementary Movie 1 ). In addition, the incoming new PM particles could attach directly to the PM that were already on the PAN nanofibres and merged together (shown in Fig. 4f and Supplementary Movie 1 ). As the capture kept going on, the PAN filters were filled with big aggregated PM particles. The junction of nanofibres had more PM accumulated and formed spherical particles in bigger sizes. Figure 4: In situ time evolution study of PM capture by PAN transparent filter. ( a – d ) In situ study of PM capture by PAN nanofibre characterized by OM showing filter morphologies at different time sequences during a continuous feed. Scale bars, 20 μm. The timescales for ( a – d ) is 0, 5, 120 and 600 s, respectively. ( e – h ) Schematics showing the mechanism of PM capture by nanofibrous filter at different time sequences. ( i ) SEM image showing the detailed morphologies of attached soft PM that formed a coating layer wrapping around the PAN nanofibre. Scale bar, 1 μm. ( j ) SEM image showing that the nanofibre junction has more PM aggregated to form bigger particles. Scale bar, 1 μm. Full size image SEM was used to characterize the detailed interaction between PM particles and PAN nanofibres, and the images are shown in Fig. 4i,j . The general capture mechanism of soft PM particle is that after being in contact with the PAN nanofibre, the PM particle would wrap around the nanofibres tightly ( Fig. 4i ), deform and finally reach to a stable spherical shape on the nanofibre. This wrapped around coating indicates that the PM particles favour the surface of PAN nanofibres so that they would like to enlarge their contact areas and bind tightly to ensure an excellent capture performance. PM chemical composition analysis To further explain the performance difference of different fibrous filters in capturing smoke PM, the composition and surface chemistry of smoke PM was investigated. 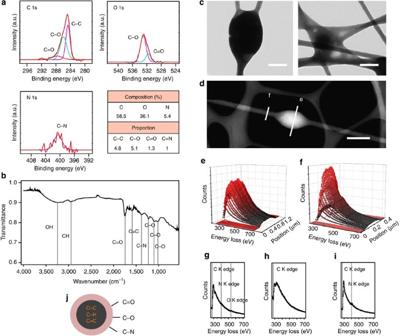Figure 5: Smoke PM composition analysis. (a) XPS characterization of PM particle showing the C 1 s, O 1 s and N 1 s peak analysis and composition ratio. (b) FTIR characterization of PM particle showing the existing functional groups. (c) TEM images showing the morphologies of PM particles captured on PAN filter. Scale bar, left, 0.5 μm; right, 1.5 μm. (d) TEM image of the PM particle captured on PAN nanofibre used for EELS analysis. Scar bar, 1 μm. (e,f) EELS data of position (e) and (f) corresponding to PM particle and PAN fibre. (g–i) Extracted EELS data on different positions: (g) surface of PM particle; (h) bulk of PM particle and (i) PAN fibre. (j) Schematic showing PM particle compositions with nonpolar functional groups (C–C, C–H and C=C) inside and polar functional groups (C=O, C–O and C–N) outside. Figure 5a shows the X-ray photoelectron spectroscopy (XPS) characterization of PM. XPS only detected the surface element composition (~5 nm in depth) of the smoke PM. It is shown that the C 1-s signal comprises three major peaks at 284.7, 285.9 and 286.6 eV, corresponding to C–C, C–O and C=O bonds. The O 1-s peaks support the results of C 1-s peaks and show the present of C–O and C=O at 533.1 and 531.9 eV, respectively. Besides these elements, a small proportion of N is present on the surface of smoke particle, which is shown at the peak of 400.8 eV of N 1 s. The overall results show that C, O and N are the three elements present on smoke PM surface and their ratio is 58.5%, 36.1% and 5.4%, respectively. The functional groups are C–C, C–O, C=O and C–N with a ratio of 4.8:5.1:1.3:1. The bulk composition of smoke PM was characterized by Fourier transform infrared spectroscopy (FTIR) and the spectra are shown in Fig. 5b . The main peaks are at ~3,311, 2,291, 1,757, 1,643, 1,386, 1,238, 1,118 and 1,076 cm −1 , which indicated the existence of O–H, C–H, C=O, C=C, C–N and C–O (last three peaks) functional groups. In addition, energy-dispersive X-ray spectroscopy (EDX) characterization showed same composition of C, N and O in PM particles (shown in Supplementary Fig. 6 ). The XPS, FTIR and EDX analyses show consistent results of the smoke composition that contains mostly organic carbon with functional groups of different polarities such as alkanes, aldehyde and so on. The functional groups of high polarities, such as C–O, C=O and C–N, are mainly distributed on the outer surface of the particles. To further demonstrate the functional group distributions across the PM particle, transmission electron microscopy (TEM) and electron energy loss spectroscopy (EELS) are used to characterize the smoke PM captured on PAN fibre. Figure 5c shows the morphologies of PM attached to the PAN fibres. The PM particles have a sticky amorphous carbon-like morphology with the cores containing some condensed solids, while the outer surfaces containing light organic matters. EELS was used to measure the energy loss across the PM attached to PAN fibre ( Fig. 5d,e ) and bare PAN fibre ( Fig. 5d,f ). The result shows that at the PM particle, the chemical contents change with position. By scanning the beam from one end of the PM to the other end, the peaks of the C K edge (284 eV), the N K edge (401 eV) and the O K edge (532 eV) were first shown at the outer surface of the PM (shown in Fig. 5g ). As the beam moved to the centre of the PM, the N K edge and O K edge signals diminished and only the C signal was present (shown in Fig. 5h ). At last, as the position moved to the outer surface again, the N K edge (401 eV) and O K edge (532 eV) peaks showed up again. As control, the EELS signal of the PAN fibre showed the same signal all across the whole fibre with C K edge (284 eV) and N K edge (401 eV), which matches the chemical composition of the PAN polymer (shown in Fig. 5i ). This indicates again that the polar functional groups that contain O and N (C–O, C=O and C–N) are mostly present on the outer surface of PM accompanied by some nonpolar functional group such as alkanes (shown in Fig. 5j ). This is consistent with the result that polymer air filters with higher dipole moments have higher PM capture efficiencies. Because the polar functional groups such as C–O, C=O and C–N were present at the outer surface of the PM particles, polymers with higher dipole moment can have stronger dipole–dipole and induced-dipole intermolecular forces so that the PM capture efficiency is higher. Figure 5: Smoke PM composition analysis. ( a ) XPS characterization of PM particle showing the C 1 s, O 1 s and N 1 s peak analysis and composition ratio. ( b ) FTIR characterization of PM particle showing the existing functional groups. ( c ) TEM images showing the morphologies of PM particles captured on PAN filter. Scale bar, left, 0.5 μm; right, 1.5 μm. ( d ) TEM image of the PM particle captured on PAN nanofibre used for EELS analysis. Scar bar, 1 μm. ( e , f ) EELS data of position ( e ) and ( f ) corresponding to PM particle and PAN fibre. ( g – i ) Extracted EELS data on different positions: ( g ) surface of PM particle; ( h ) bulk of PM particle and ( i ) PAN fibre. ( j ) Schematic showing PM particle compositions with nonpolar functional groups (C–C, C–H and C=C) inside and polar functional groups (C=O, C–O and C–N) outside. Full size image PAN transparent air filter long-term performance The long-term performance of the transparent filter was evaluated using a PAN filter with a transmittance of ~75% under the condition of hazardous level equivalent to the PM 2.5 index >300 and a mild wind condition (<1 miles per hour). The performance is shown in Fig. 6a . After 100 h, the PAN filter still maintained a high PM 2.5 and PM 10–2.5 removal efficiency of 95–100% and 100%, respectively, and the pressure drop only increased slightly from ~2 to ~5 Pa. The SEM images in Fig. 6b,c showed the morphologies of PAN nanofibrous filter after 100-h test. The PM particles captured were aggregated and formed domains of very large particles of 20–50 μm. No detachment of PM was noticed after using clean air to blow through the used PAN filter by measuring the mass loss (within 0.006% of error bar). A separate PM adsorption test has shown that the PAN transparent filter achieved a capture of PM pollutants 10 times of the mass to the filter’s self-weight. This 10 × capability implies that the lifetime of a transparent filter with the transmittance of ~75% was expected to be above 300 h under the hazardous PM level (PM index >300). 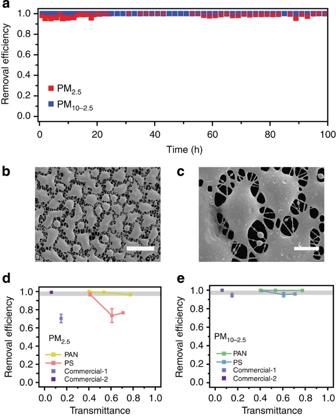Figure 6: PAN transparent filter long-term performance and field test (Beijing) performance. (a) The long-term PM2.5and PM10–2.5removal efficiencies by PAN transparent filter of 70% transmittance under continuous hazardous level of PM pollution. (b,c) SEM showing the PAN transparent air filter morphology after 100-h PM capture test. Scale bars, 50 and 10 μm, respectively. (d,e) The PM2.5and PM10–2.5removal efficiencies of PAN and PS transparent filters with different transmittance compared with commercial-1 and commercial-2 mask. Tests were performed in Beijing on 3 July 2014 under air-quality condition of PM2.5index >300. Error bar represents the standard deviation of three replicate measurements. Figure 6: PAN transparent filter long-term performance and field test (Beijing) performance. ( a ) The long-term PM 2.5 and PM 10–2.5 removal efficiencies by PAN transparent filter of 70% transmittance under continuous hazardous level of PM pollution. ( b , c ) SEM showing the PAN transparent air filter morphology after 100-h PM capture test. Scale bars, 50 and 10 μm, respectively. ( d , e ) The PM 2.5 and PM 10–2.5 removal efficiencies of PAN and PS transparent filters with different transmittance compared with commercial-1 and commercial-2 mask. Tests were performed in Beijing on 3 July 2014 under air-quality condition of PM 2.5 index >300. Error bar represents the standard deviation of three replicate measurements. Full size image Performance of the transparent air filters in a field test In order to study the efficacy of our filters in a real polluted air environment, we carried out a field test on 3 July 2014 in Beijing, China. On the basis of a recent study [29] , the PM 2.5 in Beijing has 40.7% of organic matters, which is similar to our experimental condition. The PM 2.5 concentration on that day was at a hazardous level equivalent to a PM 2.5 index >300. The results are shown in Fig. 6d,e . PAN filters with transmittance ~77%, ~54%, ~40% achieved PM 2.5 and PM 10–2.5 removal efficiencies of 98.69%, 99.42%, 99.88% and 99.73%, 99.76%, 99.92%, respectively. For comparison, a PS filter, which showed lower removal of smoke PM, consistently showed lower removal of PM 2.5 and PM 10–2.5 in the field test, of 76.61%, 73.50%, 96.76% and 95.91%, 95.17%, 99.44% at transmittance of 71%, 61%, 41%, respectively. In addition, commercial masks commercial-1 and commercial-2 with PP fibres (images shown in Supplementary Fig. 5 ) were tested for comparison. Commercial-1 showed much lower PM 2.5 and PM 10–2.5 removal of 70.40% and 94.66%, respectively. Commercial-2 showed comparable removal efficiencies of PM 2.5 (99.13%) and PM 10–2.5 (99.78%), although it is essentially not transparent (transmittance 6%). Hence, PAN showed the best performance as a transparent filter. Performance under different humidity and wind force On the basis of the real weather situation, wind force and humidity were also taken into consideration and the results are shown in Supplementary Figs 7 and 8 . The PAN fibrous filter with the transmittance of ~73% was tested at different wind force representing calm (0.21 m s −1 ), light breeze (3.12 m s −1 ), gentle breeze (5.25 m s −1 ) and fresh wind (10.5 m s −1 ) conditions. The removal efficiencies under all cases were >96.00% and showed an increasing trend of removal efficiency to wind velocity, which could be due to the increase in PM particle rejection. This is consistent with other studies [15] . For PM capture under extreme humid conditions (45% humidity and 30% humidity), the results showed that humidity helps PAN and PS with the transmittance of ~70% to achieve better PM capture, especially for PS that increased from 37.08 to 95.59%. This is because the ambient water content increased the capillary force between the PM particles and PS nanofibres during PM attachment. However, for PVP and PVA, because of their solubility in water, under extreme humid conditions, the filters were damaged significantly resulting in no detectable removal. Still under humid condition, PAN transparent filters showed the best performance. We have demonstrated that electrospun PAN nanofibres can be highly effective transparent PM filters because of its small fibre diameter and surface chemistry. Such nanofibrous filters can shut off PM from entering the indoor environment, maintain natural ventilation and preserve the optical transparency when installed on windows. An electrospun PAN transparent air filter with a transmittance of ~75% can be used under a hazardous PM 2.5 level for as long as 100 h with efficiency maintained at 95–100%. This high particle removal efficiency has also been proven by a field test in Beijing, showing the practical applicability of our transparent filters. We believe that our transparent air filter can be used as a stand-alone device or incorporated with existing masks or HEPA filters to achieve a healthier indoor living environment. Electrospinning The solution system for the polymers used in this work is 6 wt% PAN (MW=1.5 × 10 5 g mol −1 , Sigma-Aldrich) in dimethylformamide (EMD Millipore), 7 wt% polyvinylpyrrolidone (MW=1.3 × 10 6 g mol −1 , Acros) in ethanol (Fisher Scientific), 10 wt% polyvinyl alcohol (MW=9.5 × 10 4 g mol −1 , Sigma-Aldrich) in distilled water and 6 wt% polystyrene (MW=2.8 × 10 5 g mol −1 , Sigma-Aldrich) in dimethylformamide together with 0.1 wt% of myristyltrimethylammonium bromide (Acros). The polymer solution was loaded in a 1-ml syringe with a 22-gauge needle tip, which is connected to a voltage supply (ES30P-5W, Gamma High Voltage Research). The solution was pumped out of the needle tip using a syringe pump (KD Scientific). The fibre glass wire mesh (New York Wire) was sputter-coated (AJA International) with ~150 nm of copper on both sides and was grounded to collect the electrospun nanofibres. The wire diameter was 0.011 inch, and the mesh size was 18 × 16. The electrospun nanofibres would lie across the mesh hole to form the air filter, similar to previous reports [26] , [27] , [30] . The applied potential, the pump rate, the electrospinning duration and the needle-collector distance were carefully adjusted to control the nanofibre diameter and the packing density. Optical transmittance measurement The transmittance measurement used a xenon lamp (69911, Newport) as the light source, coupled with a monochromator (74125, Newport) to control the wavelength. An iris was used to trim the beam size to ~5 mm × 5 mm before entering an integrating sphere (Newport) for transmittance measurement. A photodetector (70356, Newport) was inserted into one of the ports of integrating sphere. The photodiode is connected to lock-in radiometry system (70100 Merlin, Newport) for photocurrent measurement. The samples were placed in front of the integrating sphere; therefore, both specular transmittance and diffuse transmittance were included. For air filters coated on copper wire mesh, a clean copper wire mesh with the same geometry was used as a reference. For self-standing filters, ambient air was used for reference. The transmittance spectrum was then weighted by AM1.5 solar spectrum from 400 to 800 nm to obtain the average transmittance. PM generation and efficiency measurement For all performance tests unless mentioned otherwise, model PM particles were generated from incense smoke by burning. The smoke PM particles have a wide size distribution from <300 nm to >10 μm, with the majority of particles being <1 μm. The inflow concentration was controlled by diluting the smoke PM by air to a hazardous pollution level equivalent to the PM 2.5 index >300. PM particle number concentration was detected with and without filters by a particle counter (CEM) and the removal efficiency was calculated by comparing the number concentration before and after filtration. In the rigid PM capture test, dust PM particles were fabricated by grinding soil particles using a ball mill to submicron sizes. The pressure drop was measured by a differential pressure gauge (EM201B, UEi test instrument). Unless mentioned, the wind velocity used in the efficiency test was 0.21 m s −1 and the humidity was 30%. Characterization The SEM images and EDX were taken by FEI XL30 Sirion SEM with an acceleration voltage of 5 kV for imaging and 15 kV for EDX collection. The TEM images and EELS data were collected with an FEI Titan TEM with the acceleration voltage of 300 kV. The XPS spectrum was collected using the PHI VersaProbe Scanning XPS Microprobe with an Al Kα source. The FTIR spectrum was measured using the Bruker Vertex 70 FTIR spectrometer. How to cite this article: Liu, C. et al . Transparent air filter for high-efficiency PM 2.5 capture. Nat. Commun. 6:6205 doi: 10.1038/ncomms7205 (2015).